Highly sensitive sulphide mapping in live cells by kinetic spectral analysis of single Au-Ag core-shell nanoparticles Hydrogen sulphide (H 2 S) is a gaseous signalling agent that has important regulatory roles in many biological systems but remains difficult to measure in living biological specimens. Here we introduce a new method for highly sensitive sulphide mapping in live cells via single-particle plasmonic spectral imaging that uses Au-Ag core-shell nanoparticles as probes. This strategy is based on Ag 2 S formation-induced spectral shifts of the nanoprobes, which is not only highly selective towards sulphide but also shows a linear logarithmic dependence on sulphide concentrations from 0.01 nM to 10 μM. A theoretical model was established that successfully explained the experimental observations, suggesting that the local sulphide concentration as well as its oscillations can be determined indirectly from kinetic measurements of the spectral shifts of the nanoprobes. We demonstrated for the first time the real-time mapping of local variations of sulphide levels in live cells with nM sensitivity. Hydrogen sulphide (H 2 S), traditionally considered a toxic gas with a rotten egg smell, has been recognized as an endogenous gasotransmitter with importance comparable to nitric oxide (NO) and carbon monoxide (CO), and has attracted increasing attention in recent years [1] , [2] , [3] , [4] . H 2 S equilibrates with aqueous sulphides (HS − and S 2− ) in biological environments and has vital roles in various physiological and pathological processes, including vasorelaxation [5] , angiogenesis [6] , cerebral microcirculation [7] , neurotransmission [8] , [9] , inflammation [10] , apoptosis [11] , insulin signalling inhibition [12] , oxygen sensing [13] and energy production in mitochondria [14] . Meanwhile, the H 2 S levels are related to a number of diseases, such as Down syndrome [15] , Alzheimer disease [16] , hyperglycaemia [17] , ischaemia [18] and so on. To elucidate the complex behaviours of H 2 S in both healthy and disease states, it is crucial to measure H 2 S distribution in biological systems in real time. Indeed, conventional assays using colorimetric analysis [19] , electrochemical analysis [20] , [21] and gas chromatography [22] are currently available to determine H 2 S concentrations in processed samples, such as homogenized tissues, cell lysates or blood serum. During the past several years, several research groups have developed sulphide-responsive fluorescent organic molecules to detect H 2 S in live cells and have achieved selective intracellular sulphide imaging with limits of detection of 1–10 μM (refs 23 , 24 , 25 , 26 , 27 , 28 ). Although most publications suggest that the average endogenous H 2 S level is in the μM range, much lower sulphide concentrations have been reported [29] . More importantly, the anabolism and catabolism of cellular sulphide are known to be rapid, which means that the sulphide concentration could fluctuate continuously from as high as sub-mM during its explosive production to as low as a few nM after its rapid consumption [30] . However, almost all existing H 2 S-sensing methods are based on some irreversible stoichiometric reaction between the probe and sulphide species [23] , [24] , [25] , [26] , [27] , [28] and cannot be utilized to monitor the dynamics of sulphide generation and elimination inside cells, especially at the single-molecule level. Therefore, more sensitive methods that are capable of following time-dependent changes in H 2 S concentrations over a large dynamic range are needed for in-depth studies of this gaseous transmitter. Plasmonic nanoparticles (PNPs) have long been utilized for chemical and biological sensing [31] , owing to their unique size, shape and composition as well as local environment-dependent optical properties [32] , [33] . Compared with fluorescent organic molecules, PNPs are very bright, photostable and easy to prepare. The scattering cross-section of a 54 × 14-nm gold nanorod (AuNR) at its localized surface plasmon resonance (LSPR) wavelength, for example, is ~10 5 times that of a fluorophore, making large single PNPs and their spectral changes readily observable with dark-field microscopy [34] , [35] . In addition to high sensitivity, like other single-molecule spectroscopy techniques, single PNP probes and imaging platforms provide much improved spatiotemporal resolution compared with bulk measurements. These all facilitate in situ investigations of biological processes and localized chemical reactions [36] , [37] . In this study, we present an indirect, ‘integrative’ approach for kinetic mapping of sulphide in live cells by using single-particle spectral imaging with single gold nanorod-silver (AuNR-Ag) core-shell PNPs as probes. In this plasmonic nanoprobe, the Ag shell acts as the sensing agent that reacts with the sulphide, and the AuNR core has the role of the signal reporter, whose spectrum shifts to longer wavelengths when Ag 2 S forms. Although the Ag 2 S formation reaction is irreversible, as is the case with most reported H 2 S-sensing reactions, the present study demonstrates both experimentally and theoretically that the reaction rate, and therefore, the rate of the induced spectral shifts of the PNP probes are correlated with the surrounding sulphide concentration. As a result, local intracellular sulphide concentrations and their variations were able to be determined in real time with nM sensitivity over a dynamic range of six orders of magnitude. To our knowledge, this is the first time that an intracellular gaseous transmitter has been monitored using single PNPs as optical probes. Sulphide sensing in bulk solution It is well known that in the presence of oxygen, sulphide ions selectively and quickly react with Ag atoms to generate Ag 2 S at room temperature [38] , [39] , 4Ag+2S 2− +O 2 +2H 2 O→2Ag 2 S+4OH − Because the refractive indices of Ag (~0.17) and Ag 2 S (~2.2) are substantially different [40] , [41] , the formation of Ag 2 S on an Au-Ag core-shell nanoparticle surface would result in its LSPR maximum shifting to a longer wavelength. AuNR is chosen as the core material because, as reported in the literature [34] , [42] , AuNRs with large aspect ratios, and thus LSPR maxima at long wavelengths, are highly sensitive to local refractive index variations. Accordingly, this AuNR-Ag nanoprobe exhibits a detectable colour change or redshift in its extinction spectrum even in the presence of a miniscule amount of sulphide, an advantage that could be utilized for sensitive and selective sulphide sensing. 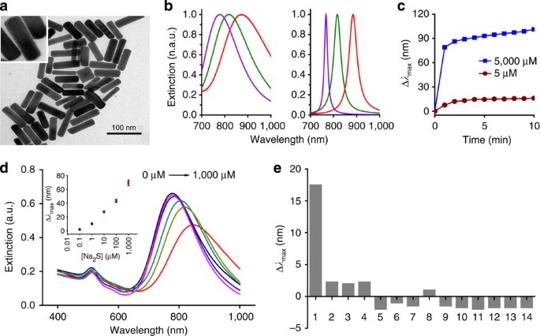Figure 1: Sulphide sensing in bulk solution with AuNR-Ag core-shell nanoprobes. (a) TEM characterization of AuNR-Ag nanoprobes with a 74 × 19-nm AuNR core and a 2.1-nm Ag shell. (b) Experimental (left) and DDA-simulated (right) LSPR spectra of AuNR (green), AuNR-Ag (purple) and AuNR-Ag2S nanoparticles. (c) Extinction spectra and Δλmaxshifts (insert) of ~50 pM PNP solution immediately after adding 0.1, 1, 10, 100 and 1000 μM of Na2S. (d) Time courses of Δλmaxincrease with the addition of 5 μM and 5 mM Na2S. (e) Selectivity for biothiols, inorganic sulphur ions and other anions. Their concentration is 25 μM unless indicated otherwise. Legend: 1, Na2S (5 μM); 2, cysteine (5 mM); 3, glutathione (5 mM); 4, Na2S2O3; 5, Na2SO3; 6, KSCN; 7, NaCl; 8, NaBr; 9, NaI; 10, NaNO2; 11. NaNO3; 12, CH3COONa; 13, Na3PO4; 14, Na2CO3. Figure 1 shows the bulk performance of AuNR-Ag PNPs having a 74 × 19-nm AuNR core and a 2.1-nm Ag shell. The longitudinal peak ( λ max ) of their LSPR spectrum occurs at 779 nm originally but shifts to longer wavelengths after addition of Na 2 S (as an aqueous H 2 S source). The λ max change (Δ λ max ) of the PNP solution (~50 pM) increases with Na 2 S concentration, and a limit of detection of 0.1 μM is achieved. The time courses of Δ λ max after adding either 5 mM or 5 μM Na 2 S to the PNP solution indicate that the PNP responds rapidly to both low and high sulphide concentrations. Because the concentrations of biothiols, such as cysteine and glutathione, in biological specimens are at mM levels [43] , [44] , the selectivity of the sulphide nanoprobe in the presence of glutathione and cysteine was tested. The spectral shifts of the PNPs induced by 5 mM of either biothiol are only ~2 nm, which is negligible compared with that induced by 5 μM sulphide. We also examined the responses of the nanoprobes towards inorganic sulphur ions (S 2 O 3 2− , SO 3 2− , SCN − ) and other anions (NO 3 − , NO 2 − , Cl − , Br − , I − , CH 3 COO − , PO 4 3− , CO 3 2− ). Because the solubility of Ag 2 S (pKsp=50.83) is much lower than other Ag compounds, no comparable LSPR responses from other species were detected even though their concentrations were much higher. Figure 1: Sulphide sensing in bulk solution with AuNR-Ag core-shell nanoprobes. ( a ) TEM characterization of AuNR-Ag nanoprobes with a 74 × 19-nm AuNR core and a 2.1-nm Ag shell. ( b ) Experimental (left) and DDA-simulated (right) LSPR spectra of AuNR (green), AuNR-Ag (purple) and AuNR-Ag 2 S nanoparticles. ( c ) Extinction spectra and Δ λ max shifts (insert) of ~50 pM PNP solution immediately after adding 0.1, 1, 10, 100 and 1000 μM of Na 2 S. ( d ) Time courses of Δ λ max increase with the addition of 5 μM and 5 mM Na 2 S. ( e ) Selectivity for biothiols, inorganic sulphur ions and other anions. Their concentration is 25 μM unless indicated otherwise. Legend: 1, Na 2 S (5 μM); 2, cysteine (5 mM); 3, glutathione (5 mM); 4, Na 2 S 2 O 3 ; 5, Na 2 SO 3 ; 6, KSCN; 7, NaCl; 8, NaBr; 9, NaI; 10, NaNO 2 ; 11. NaNO 3 ; 12, CH 3 COONa; 13, Na 3 PO 4 ; 14, Na 2 CO 3 . Full size image Sulphide detection via single-particle spectral imaging Although the PNP probes have performed as well as the fluorescent probes reported previously [23] , [24] , [25] , [26] , [27] , [28] , due to the ensemble average effect, bulk measurements are intrinsically not as sensitive as single-particle measurements. The AuNR-Ag PNP with a 2.1-nm thick silver shell, for example, contains ~6 × 10 5 silver atoms, which translates to ~30 μM Ag for a ~50 pM PNP solution. Thus, if the target sulphide concentration in the PNP solution is too low (for example, <0.1 μM), the total amount of Ag 2 S formation would not be enough to induce appreciable Δ λ max shifts for all PNPs. However, if the concentration of PNPs is reduced too much to allow more fractional coverage of Ag 2 S on each PNP, the overall optical response will not have a large enough signal-to-noise-ratio to be detected by ultraviolet–vis spectrometers. This dilemma can be resolved by monitoring the spectral shifts of individual PNPs separately using single-particle spectroscopy. Because each AuNR-Ag NP functions as an independent sulphide probe, no minimum concentration of PNPs is required. The effective ‘detection volume’ of every nanoprobe is, thus, enlarged, making it possible to accumulate or react with more sulphides locally to achieve a lower detection limit. The imaging method utilized in the present study, which was previously developed in our laboratory, is a high-throughput single-particle dark-field spectral imaging technique [45] , in which a transmission grating beam splitter (TGBS) is placed in the light collection path ( Supplementary Fig. S1 ). The TGBS splits the scattering light emitted from each PNP into a zero-order image of a focused spot and a first-order image of a long streak, and the peak-to-peak distance (after Gaussian fitting) between the spot and the streak is proportional to λ max of the particle, as dictated by Bragg diffraction. Compared with a commercial spectrograph equipped with an entrance slit, this slit-less technique can follow the spectral shifts of multiple particles or even moving particles simultaneously. To match the optimal spectral response window of the CCD camera, we prepared AuNR-Ag NPs with a 3-nm Ag shell ( λ max =622 nm, Supplementary Fig. S2 ) as the single PNP probe used in all single-particle experiments. 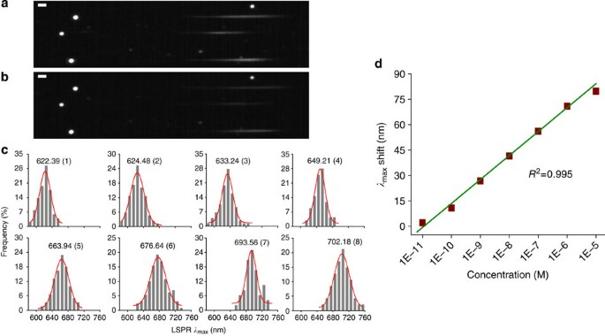Figure 2: Ultrasensitive sulphide sensing with single-particle dark-field spectral imaging. Typical single-particle spectral images (a) before and (b) after adding Na2S; a redshift is depicted as the displacement of the first-order streak towards the right. Scale bar, 2 μm. (c) Distribution of LSPR peak wavelengths after adding (1) 0 nM, (2) 0.01 nM, (3) 0.1 nM, (4) 1 nM, (5) 10 nM, (6) 100 nM, (7) 1 μM and (8) 10 μM Na2S. Over 100 particles were counted in each case. (d) The centre of theλmaxdistribution as a function of Na2S concentration added. Figure 2a display typical single-particle spectral images before and after adding Na 2 S, respectively. The separations between the first-order images and the corresponding zero-order images clearly increase with Ag 2 S formation. To investigate their sensitivity and dynamic range, we immersed single PNP probes, which were immobilized on a glass substrate, in Na 2 S solutions of different concentrations for 30 min and recorded their resulting spectral images. By Gaussian fitting the first-order streaks from randomly selected nanoprobes at each Na 2 S concentration, a Gaussian-shaped distribution of λ max values was obtained ( Fig. 2c ). All distributions were ~30 nm in width and appeared uncorrelated with Ag 2 S formation, suggesting that the difference in λ max values at the same concentration can be attributed to variations in the aspect ratios and silver shell thicknesses of single nanorods. We note that these single-particle experiments were performed with Na 2 S water solution, but due to the high selectivity of the nanoprobes, the results were nearly the same when 150 mM NaCl and 5 mM cysteine or glutathione were also present ( Supplementary Fig. S3 ). The relationship between the mean values of λ max distributions and Na 2 S concentrations is plotted in Figure 2d . An ~2-nm shift in the λ max distribution is observed when the single NP probes are exposed to a solution of just 0.01 nM Na 2 S. Amazingly, the mean Δ λ max value apparently scales up linearly with the logarithm of the applied sulphide concentration from 0.01 nM to 10 μM for six orders of magnitude. As far as we know, such a large dynamic range has never been reported for spectrally responsive single-molecule or single-particle probes. Figure 2: Ultrasensitive sulphide sensing with single-particle dark-field spectral imaging. Typical single-particle spectral images ( a ) before and ( b ) after adding Na 2 S; a redshift is depicted as the displacement of the first-order streak towards the right. Scale bar, 2 μm. ( c ) Distribution of LSPR peak wavelengths after adding (1) 0 nM, (2) 0.01 nM, (3) 0.1 nM, (4) 1 nM, (5) 10 nM, (6) 100 nM, (7) 1 μM and (8) 10 μM Na 2 S. Over 100 particles were counted in each case. ( d ) The centre of the λ max distribution as a function of Na 2 S concentration added. Full size image Sulphide concentration determination from PNP spectral shift rates To understand the underlying mechanism, we set out to study the relationship between Δ λ max and C S,NP , the sulphide concentration one AuNR-Ag core-shell PNP consumes to produce Ag 2 S on its surface. From theoretical derivations ( Supplementary Note 1 ), we can tell that Δ λ max is proportional to the local refractive index variation, Δ n (refs 32 , 46 ), which is further proportional to the molar fraction of Ag 2 S formed in the silver shell, f = C S,NP /( C Ag,0 -C S,NP ), where C Ag,0 is the total concentration of Ag atoms available. Supplementary Figure S4 plots the calculated Δ λ max as a function of C S,NP . It can be seen that while the dependence is not linear, it is by no means a logarithmic relationship. This is reasonable because C Ag,0 is a constant, and the maximum C S,NP value is limited regardless of the external sulphide concentration, . Therefore, there must be a kinetic equilibrium between the external Na 2 S concentration applied, C S,0 , and the effective concentration of sulphide capable of reacting with the silver shell, C S,eff . When C S,0 is very small, there is a large fraction of unreacted Ag, the silver shell would act like a sponge and accumulate sulphide extensively, making C S,eff larger than C S,0 . When C S,0 is large, a substantial amount of Ag 2 S forms quickly to cover the entire silver shell surface and hinder Na 2 S in the solution from reacting with Ag atoms buried under the Ag 2 S cover, so the apparent C S,eff could be much smaller than C S,0 . It is important to note that to maintain the dynamic balance of the chemical potential of the sulphides reachable to the nanoprobe, C S,eff must be equal to the sum of the concentration of sulphide in the form of Ag 2 S, , and the concentration of free sulphide accessible to the Ag atoms. A reasonable approximation for such a kinetic equilibrium is a Freundlich-absorption relationship, C S,eff = KC S,0 (1/ p ) , where K and p are both system-related constants [47] . The p -value would be >1.0 when C S,0 is small and be <1.0 when C S,0 is very large. On the other hand, from the viewpoint of reaction kinetics, Ag 2 S formation on the PNP surface can be described by a pseudo first-order reaction with O 2 in excess (in biological systems, the concentration of dissolved O 2 is generally in the sub-mM to μM range, which is much larger than the effective concentration of sulphide C S,eff in the tens of nM range that actually participated in the reaction) where is the effective concentration of free sulphide, and k obs is the observed reaction rate. Just as is a corrected form of the Na 2 S concentration applied, k obs should be the corrected form of the actual reaction rate constant, k , for the silver-sulphide reaction. It is because the silver shell contains multiple layers of silver atoms. Increasing the Ag 2 S fraction not only reduces the availability and accessibility of free Ag atoms but also makes the collisions and reactions between silver atoms and sulphide ions more difficult and less efficient. Thus, k obs can be corrected to (ref. 48 ), where A is a pre-exponential Arrhenius factor, and a is the site hindrance factor related to Ag 2 S generated on the PNP surface. The solution to the above equations is ( Supplementary Note 2 ): With C Ag,0 and k as constants and C S,eff assuming to be a constant (for simplicity), C Ag2S , C S,NP and Δ λ max as a function of time can be calculated on the basis of equation 2 to either fit or be compared with the experimental data obtained when specific Na 2 S concentrations are applied. 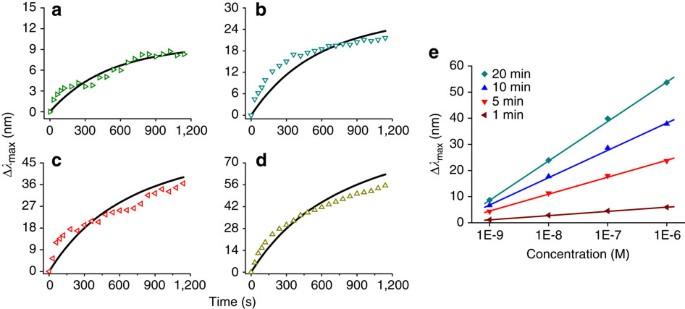Figure 3: PNP spectral shift rate varies as a function of sulphide concentration. Measured (hollow triangles) and calculated (black lines) time-dependent spectral shifts of four single AuNR-Ag nanoprobes exposed to constant concentrations of 1 nM (a), 10 nM (b), 100 nM (c) and 1 μM (d) Na2S. (e) Calculated Δλmaxvalues at various time points as a function of applied Na2S concentration. Figure 3a–d show both measured and calculated time-dependent spectral shifts of four single AuNR-Ag NPs when they were exposed to constant concentrations of 1 nM, 10 nM, 100 nM and 1 μM Na 2 S, respectively. The experimental results show that in all cases, Δ λ max increase rapidly initially and then slow down. While the applied Na 2 S concentrations differ by as much as 1,000 times, the difference in Δ λ max , even at the longest time point recorded ( t =20 min), is less than 10 times. To fit these measured results with the above equations, the p -value is adjusted individually to obtain the closest fit for each Na 2 S concentration. From the P -values obtained, we determined C S,eff to be 4.2 nM, 12 nM, 17 nM and 25 nM when the bulk Na 2 S concentrations are 1 nM, 10 nM, 100 nM and 1 μM, respectively. As expected, there is a sulphide accumulation effect at low Na 2 S concentrations (1 nM) and a sulphide hindrance effect at high Na 2 S concentrations (100 nM and 1 μM). Notice that because we cannot measure the exact effective volume or the ‘reachable range’ of a PNP probe, the values of C Ag,0 , k , p as well as C S,eff , or whether the particle accumulates or hinders Ag 2 S formation, are only relative. In other words, C S,eff is only conceptually significant in the present study, and more rigorous simulations are required to reveal whether this entity is quantitatively valid. Nevertheless, the fits to the experiments at all Na 2 S concentrations and the trends of the corresponding C S,eff values are reliable, as they are bound by actual measurements. Importantly, when we plot the calculated Δ λ max values versus the logarithm of applied Na 2 S concentration at every time point, a good linear dependence is always obtained ( Fig. 3e ). This is consistent with the experimental results shown in Figure 2c , further demonstrating that our theoretical model is a rational explanation of the experimental observations. Figure 3: PNP spectral shift rate varies as a function of sulphide concentration. Measured (hollow triangles) and calculated (black lines) time-dependent spectral shifts of four single AuNR-Ag nanoprobes exposed to constant concentrations of 1 nM ( a ), 10 nM ( b ), 100 nM ( c ) and 1 μM ( d ) Na 2 S. ( e ) Calculated Δ λ max values at various time points as a function of applied Na 2 S concentration. Full size image One consequential implication here is that through dynamic equilibrium between C S,0 and C S,eff or the Freundlich-absorption relationship, the sulphide PNP probes effectively ‘project’ external sulphide concentrations that span widely over several orders of magnitude to a narrow concentration range of surface-bound sulphide (for example, 0–30 nM, as shown in Supplementary Fig. S4 ) that matches the detectable range of the probe’s spectral response, although at the cost of reduced sensitivity and delayed responses to concentration changes. If such a dynamic equilibrium is established quickly, a reasonable assumption given that the nanoprobe is very small and Ag 2 S formation is very fast, we can indirectly obtain local sulphide concentrations in real time by using time-dependent Δ λ max plots of single PNPs under various fixed sulphide concentrations as external calibration curves ( Fig. 4a ). 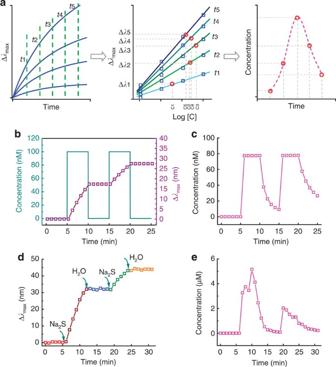Figure 4: Sulphide concentration fluctuations can be determined from PNP spectral shift rates. (a) Schematic illustration of the ‘integration sensing’ concept pertaining to the AuNR-Ag nanoprobes. Local sulphide concentrations can be obtained indirectly by using time-dependent Δλmax(increase) plots at various constant sulphide concentrations as external calibration curves. (b,c) The simulatedλmaxshift and the recovered sulphide concentration as a function of time upon a square-pulse input of 100 nM Na2S. (d,e) The experimentally measuredλmaxshift and the calculated sulphide concentration as a function of time after alternately adding 40 μl of 5 μM Na2S solution and pure water. Figure 4: Sulphide concentration fluctuations can be determined from PNP spectral shift rates. ( a ) Schematic illustration of the ‘integration sensing’ concept pertaining to the AuNR-Ag nanoprobes. Local sulphide concentrations can be obtained indirectly by using time-dependent Δ λ max (increase) plots at various constant sulphide concentrations as external calibration curves. ( b , c ) The simulated λ max shift and the recovered sulphide concentration as a function of time upon a square-pulse input of 100 nM Na 2 S. ( d , e ) The experimentally measured λ max shift and the calculated sulphide concentration as a function of time after alternately adding 40 μl of 5 μM Na 2 S solution and pure water. Full size image Notice that while the Ag 2 S formation itself is irreversible, it is the observed reaction rate on the PNP surface that is responsive to variations in sulphide concentrations in the surrounding environment. As long as free silver atoms are available, the observed Ag 2 S formation rate as well as the λ max shifting rate would increase as the external sulphide concentration increases and vice versa. Figure 4b show Δ λ max values simulated using the equations derived earlier and the calculated sulphide concentrations using Fig. 3e as the calibration curves, respectively, as a function of time upon input of a square-pulse of external sulphide. The trend observed for the recovered time-dependent variation in sulphide concentrations is very similar to that of the input, although there is some delay during the concentration reduction process because of the integrative nature of the nanoprobe. The slight deviations in the recovered sulphide concentration values are most likely due to the oversimplification of our derivations and the less accurate measurement(s) of analytical working curves, which are systematic factors that can likely be corrected with the future development of more rigorous theories and better experimental conditions. Figure 4d shows the spectral shifts measured after alternately applying 5 μM Na 2 S and pure water to an AuNR-Ag particle immobilized in a flow channel. The calculated local sulphide concentration and its variation are satisfactory ( Fig. 4e ). Therefore, this PNP nanoprobe is capable of tracking sulphide concentration fluctuations. Real-time H 2 S mapping in live cells To determine whether these single AuNR-Ag PNPs and this indirect method for sulphide analysis is applicable to live cells, we incubated the PNPs with HeLa cells. Standard assays indicate that these PNPs do not aggregate in cell culture media with serum and have almost no cytotoxicity (data not shown). After incubation for 4 h, some PNPs were found in the cytoplasm of the cells, where the PNPs appeared as bright orange spots under dark-field illumination. Because the PNPs have much higher intensities than intracellular organelles, the zero-order spots (position) and the first-order streaks (spectrum) of the nanoprobes inside the cell can be readily obtained, especially after background subtraction ( Supplementary Fig. S5 ). As a control experiment, we monitored the spectra of individual PNPs continuously for 40 min in the absence of sulphide. The variation in their λ max values was found to be ~2 nm ( Supplementary Fig. S6 ), indicating that these PNPs are highly stable spectrally within the intracellular environment. Next, Na 2 S was added to the cell culture medium to a final concentration of 0.1 μM. Time-dependent colour images and spectral variations of two single PNPs were recorded simultaneously for 40 min. 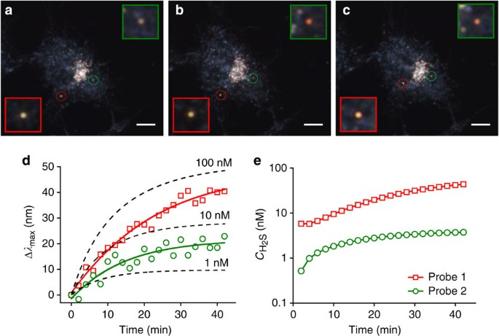Figure 5: Local variations of intracellular sulphide levels can be determined in real time. (a–c) Representative images showing the gradual colour changes of two individual PNPs after adding 0.1 μM Na2S to the cell culture medium for (a) 2 min, (b) 26 min and (c) 42 min. Scale bar, 10 μm. The red and green square inserts are enlarged images of the two circled PNPs. (d) Observed (hollow dots) and fitted (lines) time-dependentλmaxshifts of the two particles. The calculated dynamic Δλmaxshifts at 1, 10 and 100 nM adapted fromFig. 3a–dare also plotted (dashed lines) for reference. (e) Calculated time-dependent change in local sulphide concentrations surrounding the two particles according to the fitted results ind, usingFig. 3eas the external calibration curves. During this time period, as shown in Figure 5 and Supplementary Fig. S7 , the λ max of one particle (red circle, P1) redshifted by ~40 nm, while the other (green circle, P2) changed ~20 nm. Although the two AuNR-Ag particles were not exactly the same in terms of their aspect ratios (their initial λ max difference was ~20 nm), single-particle heterogeneities alone cannot account for such a large spectral response difference according to our simulations ( Supplementary Fig. S8 ). Therefore, the local sulphide concentration and its accumulations around the two particles must be different. Comparing the fitted Δ λ max plots of P1 and P2 with Δ λ max reference plots in Fig. 3 , the sulphide concentrations experienced by P1 apparently falls between 10 nM to 100 nM, while that experienced by P2 falls between 1 nM and 10 nM ( Fig. 5d ). Using the curves in Fig. 3e as external calibration curves and the Δ λ max values from data interpolations in Fig. 5d as inputs, the time-dependent local sulphide concentration increases are determined for both particles ( Fig. 5e ). From 2 min to 40 min, the apparent local concentration of sulphide experienced by P1 changes from 5.8 nM to 41.8 nM, whereas that experienced by P2 changes from 0.5 nM to 3.8 nM. These values are all smaller than the 100 nM sulphide concentration supplied externally but are reasonable for such an ‘integration sensor’. Because sulphide is highly diffusive and reactive, the large difference between P1 and P2 is most likely an indication of heterogeneous diffusion, distribution or consumption of sulphide throughout the cell. Although the indirectly measured sulphide concentrations may deviate more or less from the true values due to some systematic errors, the magnitudes as well as the trends of the calculated values are nevertheless reliable. Most previous reports regarding fluorescent sulphide probes were only able to provide static whole-cell images and reveal qualitative fluorescence intensity differences (among these images) after 15–30 min external stimulations with various sulphide concentrations in the μM range [24] , [26] , [28] , [29] To our knowledge, ours is not only the first demonstration of live cell sulphide imaging with nM sensitivity but is also the first time that local variations in intracellular sulphide levels have been tracked dynamically. Figure 5: Local variations of intracellular sulphide levels can be determined in real time. ( a–c ) Representative images showing the gradual colour changes of two individual PNPs after adding 0.1 μM Na 2 S to the cell culture medium for ( a ) 2 min, ( b ) 26 min and ( c ) 42 min. Scale bar, 10 μm. The red and green square inserts are enlarged images of the two circled PNPs. ( d ) Observed (hollow dots) and fitted (lines) time-dependent λ max shifts of the two particles. The calculated dynamic Δ λ max shifts at 1, 10 and 100 nM adapted from Fig. 3a–d are also plotted (dashed lines) for reference. ( e ) Calculated time-dependent change in local sulphide concentrations surrounding the two particles according to the fitted results in d , using Fig. 3e as the external calibration curves. Full size image In addition to sensing sulphide supplied from outside the cell, we also determined if our PNP probes could be utilized to map spatially resolved concentrations of sulphides generated inside live cells. Previous studies have demonstrated that the cystathionine β-synthase (CBS) enzyme, which is involved in H 2 S generation using cysteine and homocysteine as sulphide sources, is strongly expressed in nonconfluent HepG2 cells, but the activity of CBS is significantly decreased after the cells are treated with human insulin [49] , [50] , [51] , [52] . Thus, we adopted normal and insulin-pretreated HepG2 cells as model cells, incubated them with the PNPs, and examined whether variations in intracellular H 2 S production could be detected. 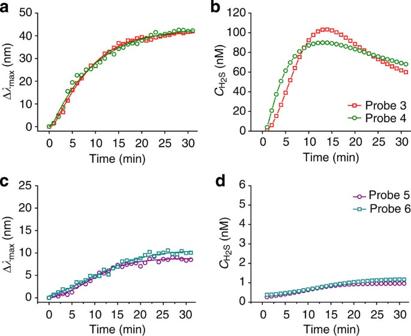Figure 6: Endogenous sulphide concentrations can be determined. Observed (hollow dots) and fitted (lines) time courses of Δλmaxshifts of representative PNPs in HepG2 cells without (a) and with (c) insulin pretreatment. Cysteine and homocysteine were used as the H2S source. Calculated real-time local H2S concentration variations for these two cases are shown inbandd, respectively. As seen in Figure 6 and Supplementary Fig. S9 , after adding cysteine and homocysteine to the cell culture medium for 30 min, the λ max shifts of two representative PNPs in the normal HepG2 cell were significantly larger than those in the cell pretreated with human insulin. The calculated intracellular H 2 S concentration around the PNPs in the normal HepG2 cells rose quickly to ~100 nM and then declined gradually ( Fig. 6b ), most likely because of an increase in the gaseous-transmitter-induced sulphide catabolism or the diffusion of sulphide into the extracellular medium. In contrast, the H 2 S concentration in the insulin-pretreated HepG2 cell increased slowly to only ~1 nM ( Fig. 6d ), consistent with the prediction that the CBS activity as well as H 2 S production was greatly reduced. In the negative control experiment, no PNP spectral shifts were observed if cysteine and homocysteine were not added ( Supplementary Fig. S9e ). Hence, differences in endogenous H 2 S levels were successfully tracked in real time, and our AuNR-Ag core-shell PNPs can be utilized to map spatial-temporal distributions of biologically produced H 2 S inside live cells. Figure 6: Endogenous sulphide concentrations can be determined. Observed (hollow dots) and fitted (lines) time courses of Δ λ max shifts of representative PNPs in HepG2 cells without ( a ) and with ( c ) insulin pretreatment. Cysteine and homocysteine were used as the H 2 S source. Calculated real-time local H 2 S concentration variations for these two cases are shown in b and d , respectively. Full size image This study introduces a new method for highly sensitive sulphide mapping on the basis of single-particle spectral imaging using AuNR-Ag core-shell nanoparticles as probes. The integrative-Ag 2 S-formation-induced time-dependent spectral shifts of the nanoprobes are not only highly selective towards sulphide but also show a linear logarithmic dependence on sulphide concentrations at all time points. A theoretical model was established that successfully explains the experimental observations and suggests that local sulphide concentrations can be determined from kinetic measurements of spectral shifts of the nanoprobes. This model allows real-time detection of local variations of sulphide levels in live cells with nM sensitivity over a large dynamic range. Being a technique that essentially measures ‘localized concentrations’ at the single-molecule level, this integrative sensing approach, based on single PNP imaging platforms and probes, could potentially be utilized to develop highly sensitive detection methods for other small molecules or ions. Chemicals and PNP preparation Human insulin, pyridoxal 5-phosphate and polyvinyl pyrrolidone (MW=29,000) were obtained from Sigma-Aldrich. All other reagents were AR grade and were purchased from Shanghai Sinopharm. AuNR synthesis and purification procedures were adopted elsewhere [53] , [54] . The resulting AuNRs were used as seeds for the growth of AuNR-Ag NPs according to the literature with some modifications [55] . In brief, 0.8 ml of purified AuNR solution was mixed with 2.4 ml of 3% polyvinyl pyrrolidone aqueous solution, after which freshly prepared ammoniacal silver nitrate (120 μl, 1 mM) was added to the mixture while stirring, followed by addition of ascorbic acid solution (120 μl, 10 mM). Finally, the solution was placed into a water bath and kept undisturbed at 30 °C until the colour change was complete. The as-prepared PNP probes were characterized with ultraviolet–vis spectroscopy (Shimadzu UV-1800, Japan) and transmission electron microscopy (TEM, JEM 1230, JEOL, Japan). Single-particle dark-field spectral imaging The experiments employed a single-particle spectral dark-field microscope with a wavelength resolution of 1.73 nm per pixel (after calibration). The set-up was composed of a Nikon 80i optical microscope (Japan), an oil-immersion dark-field condenser (numerical aperture 1.20–1.43), a 60 × Plan Fluor objective, a TGBS (70 grooves per mm, Edmund Optics), a CoolSNAP HQ2 CCD camera (with an optimal spectral response window of 470–630 nm with quantum efficiency >60%, Roper Scientific) and an Olympus DP72 colour CCD camera. In vitro sulphide detection To detect sulphide with dark-field spectral microscopy, home-built flow channels were prepared with coverslips and double-sided adhesive tape (5 mm wide, ~40 μl total volume). Before each experiment, 20 μl of AuNR-Ag PNPs (~25 pM) was injected into a flow channel, and the PNPs were absorbed onto the glass surface by adjusting the pH of the solution. After 20 min, unabsorbed PNPs were washed away by rinsing with water three times. Then, 40 μl Na 2 S solution was injected into the channel and LSPR scattering spectral images of individual nanoparticles were recorded using the single-particle spectral microscope at different time points with an exposure time of 1 s. This process was repeated for Na 2 S solutions of various concentrations. Image analyses were performed using the ImageJ software, and LSPR spectral maxima of each nanoparticle were obtained using the peakfit code in the Matlab program. Intracellular sulphide mapping Human cervical cancer (HeLa cell) lines and human hepatoma (HepG2) cells were obtained from the American Type Culture Collection (ATCC, USA). The cells were maintained in Dulbecco’s modified Eagle’s medium (Gibco) supplemented with 10% fetal bovine serum (Gibco) at 37 °C, 5% CO 2 in a humidified atmosphere. The cells were cultured on a cleaned cover-glass in a plastic cell culture dish. Internalization of nanoprobes was realized by adding 5 μl (50 pM) of AuNR-Ag PNPs to the cell culture dish and incubating for 4 h. To study sulphide transport into the cytoplasm and to monitor intracellular sulphide in real time, the cover-glass was inverted and placed on a glass slide with a concave cavity in the centre, to which the cell culture medium containing 100 nM Na 2 S was applied. Because the redshifting rate of the PNP spectra in live cells was slow, the LSPR scattering images were recorded every 2 min with an exposure time of 2 s. To suppress CBS activity in HepG2 cells, human insulin was added (with a final concentration of 1 μM) to the cell culture medium, and the cells were incubated for 48 h. For endogenous H 2 S imaging in live cells, normal and insulin-pretreated HepG2 cells were first incubated with the PNPs for 4 h. The CBS cofactor (pyridoxal 5-phosphate, at a final concentration of 200 μM) and the sulphide source (1 mM cysteine and 1 mM homocysteine) were then added to the culture medium, and the LSPR spectra of PNPs in the HepG2 cells with or without human insulin pretreatment were monitored using single-particle dark-field spectral microscopy. To track endogenous H 2 S levels, LSPR spectral images were recorded every minute with an exposure time of 2 s. How to cite this article: Xiong, B. et al . Highly sensitive sulphide mapping in live cells by kinetic spectral analysis of single Au-Ag core-shell nanoparticles. Nat. Commun. 4:1708 doi: 10.1038/ncomms2722 (2013).